Coherent properties of single rare-earth spin qubits Rare-earth-doped crystals are excellent hardware for quantum storage of photons. Additional functionality of these materials is added by their waveguiding properties allowing for on-chip photonic networks. However, detection and coherent properties of rare-earth single-spin qubits have not been demonstrated so far. Here we present experimental results on high-fidelity optical initialization, effcient coherent manipulation and optical readout of a single-electron spin of Ce 3+ ion in a yttrium aluminium garnet crystal. Under dynamic decoupling, spin coherence lifetime reaches T 2 =2 ms and is almost limited by the measured spin-lattice relaxation time T 1 =4.5 ms. Strong hyperfine coupling to aluminium nuclear spins suggests that cerium electron spins can be exploited as an interface between photons and long-lived nuclear spin memory. Combined with high brightness of Ce 3+ emission and a possibility of creating photonic circuits out of the host material, this makes cerium spins an interesting option for integrated quantum photonics. The outstandingly long optical coherence times of rare-earth-based crystals result in efficient memories for quantum states of single photons [1] and of entangled photon pairs [2] , [3] . Even longer coherence storage times can be achieved in nuclear spin memories [4] , [5] , [6] . In these quantum memories, the quantum state of a photon is stored in an electron or nuclear spin wave created in an ensemble of spins. This type of memory is suitable for storage at a single photon level [7] and, therefore, is an essential ingredient of quantum repeaters [8] and quantum-computing protocols based on linear optics [9] . However, ensemble-based rare-earth quantum computer designs lack certain functionalities such as error correction that are essential for scalability [10] . This problem can be resolved by addressing single rare-earth spins individually. In the last 2 years, detection of several rare-earth species at a single ion level was demonstrated [11] , [12] , [13] , [14] , although no long-lasting spin coherence for single ions was demonstrated so far. In this Article, we for the first time demonstrate optically addressable rare-earth single-spin qubit in an oxide crystal, namely, cerium ion in yttrium aluminium garnet (YAG), which can be optically initialized, coherently manipulated with microwaves and read out optically. Optical isolation of a single Ce 3+ in YAG Experimentally, individual cerium ions were identified in an ultra-pure YAG crystal using confocal microscopy [13] at T ≈3.5 K (see Methods section and Supplementary Fig. 1 ). In order to improve the fluorescence collection efficiency of the microscope, a solid immersion lens (SIL) was fabricated on the surface of the sample by focused ion beam (FIB) milling. Cerium ions were excited by a frequency-doubled femtosecond Ti:sapphire laser at 460 nm matching the wavelength of the phonon-assisted absorption band of Ce 3+ in YAG. Their emission associated with the 5 d →4 f (see Fig. 1a ) transition was detected in a 475–630-nm spectral window. The image of individual cerium ions under the SIL is shown in Fig. 1b . The single nature of the photon emitter was confirmed with photon antibunching measurements as indicated in Fig. 1c . The detected emission of an individual cerium ion amounts to 60–70 × 10 3 photons s −1 . The emission spectrum of the ions is indicated in Fig. 1d , showing broadband phonon-assisted emission and a sharp zero-phonon line at 489 nm (see Fig. 1e ) characteristic for cerium ions [15] . Cerium fluorescent centres can be created in YAG crystal by ion implantation (see Fig. 1f and Methods section for the details on implantation). The yield of fluorescent cerium ions was estimated to be at least 8%. It is believed that the yield can be significantly improved by thermal annealing in a reducing atmosphere [16] . 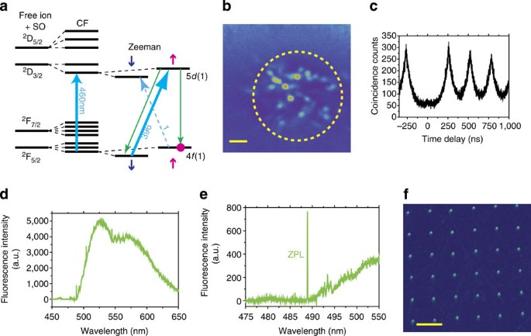Figure 1: General properties of a single Ce3+ion in YAG. (a) Electronic level structure of Ce3+ion in YAG crystal. Blue arrows pointing upwards indicate electronic transitions under laser excitation, while green arrows pointing downwards represent cerium fluorescence. Relative strengths of optical transitions between the lowest 4fand the lowest 5dspin doublets (396:1) are shown for circularly polarized excitation light propagating along theyaxis of the local Ce3+symmetry frame. External magnetic field along theydirection splits the spin doublets. Spin-up and spin-down states are indicated by short up- and down-arrows next to the corresponding energy level. (b) Confocal scan of individual cerium centres under the SIL. The scale bar is 2 μm. The dashed circle indicates boundary of the SIL. (c) Photon-correlation signal taken on a single Ce3+centre under pulsed laser excitation (see Methods section for details on antibunching measurements). The absence of the fluorescence peak at zero delay indicates single nature of the photon emitter. (d) Typical spectrum of a single cerium ion at 3.5 K. (e) Higher-resolution spectrum of Ce3+in the vicinity of its zero-phonon line (ZPL). The positions of ZPLs for distinct cerium centres are slightly different depending on the local environment of each centre. (f) Focused beam of cerium ions (300 keV) was used to create a grid of Ce3+-doped spots in YAG single crystal. The scale bar is 10 μm. Figure 1: General properties of a single Ce 3+ ion in YAG. ( a ) Electronic level structure of Ce 3+ ion in YAG crystal. Blue arrows pointing upwards indicate electronic transitions under laser excitation, while green arrows pointing downwards represent cerium fluorescence. Relative strengths of optical transitions between the lowest 4 f and the lowest 5 d spin doublets (396:1) are shown for circularly polarized excitation light propagating along the y axis of the local Ce 3+ symmetry frame. External magnetic field along the y direction splits the spin doublets. Spin-up and spin-down states are indicated by short up- and down-arrows next to the corresponding energy level. ( b ) Confocal scan of individual cerium centres under the SIL. The scale bar is 2 μm. The dashed circle indicates boundary of the SIL. ( c ) Photon-correlation signal taken on a single Ce 3+ centre under pulsed laser excitation (see Methods section for details on antibunching measurements). The absence of the fluorescence peak at zero delay indicates single nature of the photon emitter. ( d ) Typical spectrum of a single cerium ion at 3.5 K. ( e ) Higher-resolution spectrum of Ce 3+ in the vicinity of its zero-phonon line (ZPL). The positions of ZPLs for distinct cerium centres are slightly different depending on the local environment of each centre. ( f ) Focused beam of cerium ions (300 keV) was used to create a grid of Ce 3+ -doped spots in YAG single crystal. The scale bar is 10 μm. Full size image Initialization of the spin state The electronic level structure of cerium substitutional impurities in ceramic crystals is shown in Fig. 1a . The strongest transition between the ground 4 f (1) and the optically excited 5 d (1) spin doublets under σ + circularly polarized excitation is the spin flip transition |4 f (1)↓›→|4 d (1)↑›. The other three transitions are almost three orders of magnitude weaker [13] . However, decay back to the two ground states is equally probable. Repeated excitation results in efficient pumping of the ion into spin-up ‘dark’ state, thereby initializing the cerium spin. To further reveal the pumping dynamics of the cerium spin, a magnetic field of 490 G parallel to the excitation beam was applied to the sample, the excitation laser was chopped such that the cerium centre is excited with a train of pulses and the time evolution of the excited fluorescence was investigated (see Fig. 2a ). As shown in Fig. 2b , right after the circularly polarized excitation is switched on, the emission intensity is maximal determined by thermalized populations of the ground-state spin sublevels. It rapidly drops because of optical pumping into the ‘dark’ spin state. The ratio of the fluorescence intensities in the beginning of the fluorescence decay and after the spin is polarized indicates >97% fidelity of spin initialization. The fidelity of spin initialization not reaching the theoretically predicted ratio 396:1 is thought to be because of a slight ellipticity of the polarization caused by non-perfect λ /4 waveplate and polarization distortion because of the SIL. Under linearly polarized excitation, cerium emission does not depend on time indicating the absence of optical pumping. The dependence of the emission on the ellipticity of the excitation is given in Supplementary Fig. 2 . 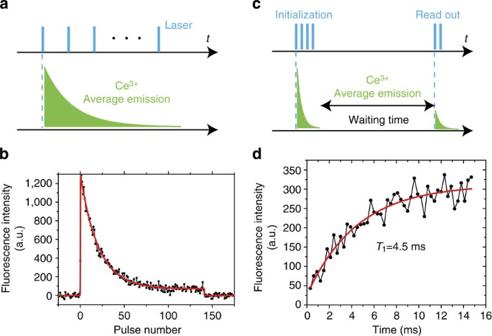Figure 2: Initialization and thermalization of Ce3+spin. (a) Schematic diagram of the laser pulse sequence used to study the initialization dynamics. The time interval between the trains was chosen to be long enough for the spin population to thermalize. The photons accumulated after each pulse in the train are summed up and they represent one point on the initialization fluorescence curve. The detailed information on the excitation pulse sequence and on the fitting procedure is given in the Methods section. (b) Dependence of the fluorescence intensity on the pulse number during initialization process. (c) Laser pulse sequence used to measure spin relaxation timeT1. The initializing pulse train is long (140 pulses) to ensure spin polarization. The readout pulse train contains only five pulses. The time interval between initializing the spin and reading it out is varied. (d) Spin relaxation curve recorded by detecting the fluorescence during readout pulse train. Inb,dred curves are the fits to the observed signals. Figure 2: Initialization and thermalization of Ce 3+ spin. ( a ) Schematic diagram of the laser pulse sequence used to study the initialization dynamics. The time interval between the trains was chosen to be long enough for the spin population to thermalize. The photons accumulated after each pulse in the train are summed up and they represent one point on the initialization fluorescence curve. The detailed information on the excitation pulse sequence and on the fitting procedure is given in the Methods section. ( b ) Dependence of the fluorescence intensity on the pulse number during initialization process. ( c ) Laser pulse sequence used to measure spin relaxation time T 1 . The initializing pulse train is long (140 pulses) to ensure spin polarization. The readout pulse train contains only five pulses. The time interval between initializing the spin and reading it out is varied. ( d ) Spin relaxation curve recorded by detecting the fluorescence during readout pulse train. In b , d red curves are the fits to the observed signals. Full size image The lifetime of the initialized spin state, T 1 , was measured by introducing the second (readout) train of laser pulses having the same circular polarization and varying the time interval between initialization and readout (see Fig. 2c ). The fluorescence recovery indicates thermalization of the spin states revealing in the spin relaxation time of T 1 =4.5 ms (see Fig. 2d ). Optical detection of Ce 3+ spin resonance The initialized spin can be manipulated by microwave radiation resonant with the spin transition of the ground 4 f (1) state. For that purpose, a microwave structure was created on the surface of the sample right next to the location of the SIL. This allowed us to record optically detected magnetic resonance (ODMR [17] ) spectra of individual cerium ions. Once the frequency of microwaves matches that of the spin transition, the population from the |4 f (1)↑› state is pumped back into |4 f (1)↓› and the overall fluorescence yield increases. A typical ODMR spectrum of a single cerium ion is shown in Fig. 3a . Linewidths of ODMR spectra are in the range of 10–15 MHz varying slightly for different cerium centres. The width of the ODMR line is determined by two factors: inhomogeneous broadening of the line because of random magnetic field produced by 27 Al nuclei and microwave power broadening. Since Ce 3+ can occupy six magnetically inequivalent sites in YAG, in general, six distinct positions of ODMR peak are possible. A combination of measured ODMR frequency and known g-tensor of the ground-state Ce 3+ spin [18] allowed us to determine the orientation of individual cerium sites. In our (110) oriented crystal, the ODMR resonances were at 640 and 1,310 MHz and four nearly degenerate ones around 1,550 MHz. For further experiments, we were choosing the centres having their local y axis (we adopted the axes assignment from the work [19] ) oriented along the magnetic field and the excitation beam (640 MHz) since for these centres the theoretical predictions for spin initialization fidelity is the best. 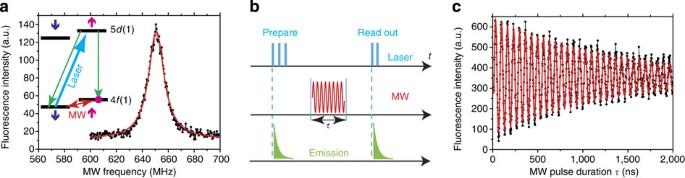Figure 3: Coherent manipulation of Ce3+spin. (a) ODMR signal of a single Ce3+ion as the frequency of microwaves (MW) is swept across the spin resonance. Inset shows level structure of the ground-state and the optically excited spin doublets. The red line is the Lorentzian fit to the observed signal. (b) Schematic diagram of Rabi measurements. (c) Spin Rabi oscillations of a single Ce3+spin. The red line is the fit to the data. The observed signal was fitted with exponentially decaying cosine function with constant offset. Figure 3: Coherent manipulation of Ce 3+ spin. ( a ) ODMR signal of a single Ce 3+ ion as the frequency of microwaves (MW) is swept across the spin resonance. Inset shows level structure of the ground-state and the optically excited spin doublets. The red line is the Lorentzian fit to the observed signal. ( b ) Schematic diagram of Rabi measurements. ( c ) Spin Rabi oscillations of a single Ce 3+ spin. The red line is the fit to the data. The observed signal was fitted with exponentially decaying cosine function with constant offset. Full size image Coherent manipulation of Ce 3+ spin The first step towards coherent manipulation of cerium electron spin is detection of Rabi oscillations under strong microwave driving. Experimentally, the circularly polarized laser excitation was chopped such that only a few tens of laser pulses are used to initialize the spin in |4 f (1)↑›. After this, a microwave pulse at resonant frequency of variable duration was applied (see Fig. 3b ). Finally, a short laser pulse train having identical circular polarization was applied to read out the population of the |4 f (1)↓› spin state. The result of the measurement is shown in Fig. 3c . The frequency of Rabi oscillations has square-root dependence on microwave power. The decay time of oscillations is longer than determined by the inhomogeneous linewidth indicating partial locking of the spin by microwaves. Dephasing of cerium spin was measured by decay of Hahn echo signal (a sequence of π /2− τ − π − τ − π /2 microwave pulses, see inset in Fig. 4a ). The result yields a value of T 2 =2 τ =240 ns, where τ is the free evolution time between π /2 and π pulses. Fast decoherence in YAG can be explained by the presence of the dense bath of 27 Al having spin of I =5/2 accompanied by large magnetic moment μ Al =3.64 μ N with μ N being nuclear magneton. Fluctuating nuclear spins produce magnetic noise at the location of Ce 3+ reducing coherence time. Theoretical analysis of the nuclear spin bath showed that the contribution of octahedrally coordinated 27 Al nuclei to decoherence is the largest (see Supplementary Methods ). 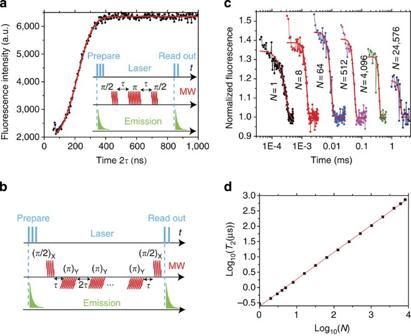Figure 4: Dynamic decoupling of Ce3+spin from spin bath. (a) Spin-echo decay shows a decoherence timeT2=240 ns. The decay is non-exponential. The red curve represents Gaussian fit to the echo signal. (b) Schematic diagram of measuring the decoherence time with CPMG decoupling sequence. After applying the firstπ/2 microwave pulse (Xπ/2 pulse) and waiting for timeτ, one applies a sequence ofπ-microwave refocusing pulses separated by 2τand phase-shifted from the Xπ/2 pulse by 90° (Yπpulses). Rotation alongy- instead ofxplane on the Bloch sphere makes the sequence robust. (c) Results of CPMG measurements for several sequences. The number of pulses for each sequence is given for the corresponding decay curve. Stretched-exponential fits to the data are shown by red curves. (d) The dependence of the coherence lifetime on the length of CPMG sequence. The red curve is the linear fit to the data points in log-log scale. The slope of 0.88 is closer to the linear dependence characteristic to nuclear spin bath rather than toN2/3characteristic to the electron spin bath. Figure 4: Dynamic decoupling of Ce 3+ spin from spin bath. ( a ) Spin-echo decay shows a decoherence time T 2 =240 ns. The decay is non-exponential. The red curve represents Gaussian fit to the echo signal. ( b ) Schematic diagram of measuring the decoherence time with CPMG decoupling sequence. After applying the first π /2 microwave pulse (X π /2 pulse) and waiting for time τ , one applies a sequence of π -microwave refocusing pulses separated by 2 τ and phase-shifted from the X π /2 pulse by 90° (Y π pulses). Rotation along y - instead of x plane on the Bloch sphere makes the sequence robust. ( c ) Results of CPMG measurements for several sequences. The number of pulses for each sequence is given for the corresponding decay curve. Stretched-exponential fits to the data are shown by red curves. ( d ) The dependence of the coherence lifetime on the length of CPMG sequence. The red curve is the linear fit to the data points in log-log scale. The slope of 0.88 is closer to the linear dependence characteristic to nuclear spin bath rather than to N 2/3 characteristic to the electron spin bath. Full size image Dynamic decoupling of Ce 3+ spin from the nuclear bath Dynamic decoupling exploiting sequences of π microwave pulses allows for an enormous increase in decoherence time [20] . Decoherence is caused by the averaging over a phase factor C ( t )=‹ e i ϕ ( t ) › the Ce 3+ spin acquires during free evolution. π pulses applied with frequency 1/ τ effectively eliminate noise spectral components ν noise <1/ τ and thus lead to lenghtening of coherence lifetime. We used Carr–Purcell–Meiboom–Gill (CPMG) microwave decoupling sequence [21] , [22] (see Fig. 4b ). The maximum number of refocusing pulses applied was 24,576. This allowed us to extend decoherence time up to 1.97 ms. The measured CPMG-echo signals shown in Fig. 4c agree well with the ones simulated by noise spectrum analysis and cluster expansion method [23] (see Supplementary Fig. 3 ). The dependence of the decoherence time on the number of CPMG pulses allows one to discriminate the influence of nuclear and electronic spin baths. The latter is composed of residual transition metal spin impurities such as Cr 3+ and Fe 3+ . Electron and nuclear spin baths have significantly different noise spectral densities. The noise of the electron spin bath is best decribed by a Lorenzian-shaped spectrum characterized by a long spectral tail. This leads to a N 2/3 depencence of the coherence time [24] , [25] . On the other hand, nuclear spin noise is characterized by a much harder cutoff leading to a linear dependence of T 2 on N . The experimentally measured dependence shown in Fig. 4d is T 2 ∝ N 0.88 indicating that both nuclear and electron spin baths lead to decoherence with former contribution prevailing. Stretched-exponential fits (exp(−( t / T 2 ) k )) to CPMG-echo signals result in exponentials k between 6 and 12 confirming the existence of hard cutoff of the nuclear spin noise spectrum as described in Supplementary Methods . These results suggest that changing the host material to a low nuclear spin one—that is, yttrium orthosilicate in which rare-earth ions show the longest coherence and population lifetimes [5] , [26] , [27] , should greately increase coherence lifetime in our single spin experiments. Changing the host material has almost no effect on the atomic-like polarization selection rules of Ce 3+ crucial for initializing its spin state. Preliminary measurements indeed show extended coherence lifetime in the excited 5 d state in yttrium orthosilicate compared with YAG (see Supplementary Fig. 4 ). An important asset of YAG and similar materials is that they are suitable for integrated photonic circuit fabrication, for example, in the form of thin films on low refractive index substrates (quartz) [28] , [29] . Subsequent FIB milling would allow for creating on-chip photonic circuits with low attenuation (1.5 dB cm −1 (ref. 28 )) for single photons, which would include waveguides, cavities and so on. This would result in technologically simple realization of an on-chip integration of cerium spin qubits and, simultaneously, in obtaining access to longer-living isolated nuclear spins magnetically coupled the electron spin of Ce 3+ . Experimental setup Optical studies of single Ce 3+ ions were performed in a home-built confocal microscope in which the crystal was mounted on a cold finger of a helium flow cryostat. An optical access was arranged through a window. The microscope objective lens of numerical apperture 0.95 was mounted inside the cryostat on a piezo nano-positioner. A toroidal permanent magnet was fixed on the objective lens to provide magnetic field parallel to the propagation direction of the excitation laser beam. The fluorescence of cerium ions was collected by the same objective lens and detected with a single photon counting avalanche photodiode (APD). To perform photon-correlation measurements, the fluorescence signal was split by a 50/50 beamsplitter and detected by two separate APDs. The signals of the two APDs were analysed by Becker and Hickl time-correlated single-photon counter card. In order to measure the emission spectra, the fluorescence was deflected by a mirror mounted on a flip mount on a grating spectrometer equipped with a cooled CCD camera. For measurements involving microwaves, a high-power MW amplifier (50 dB amplification, 30 W maximum output power) was used. The frequency of microwaves was swept by a software-controlled MW synthesizer. The microwaves were supplied to the sample by a single copper wire positioned next to the SIL. The wire was lithographically defined on the surface of the crystal and electroplated. The cross-section of the wire amounted to 20 μm wide and 10 μm high with its length being several hundred microns. The wire was electrically contacted to the microwave source on one side and to the 50-Ω-terminated drain on the other. No measures were taken to ensure impedance matching. However, the measured MW loss in the wire amounted to only 6 dB. Sample preparation In order to improve fluorescence collection efficiency, a solid immersion microlens was fabricated directly on the surface of the sample by FIB milling. The lens had a shape of half-a-sphere with the radius of 5 μm. In order to perform spin manipulations with microwaves, a copper microwave structure was created next to the location of the SIL by lithographic means. Even though the microwave structure was not impedance-matched to the outer MW network, the measured overall MW loss amounted to only 6 dB. Details on initialization of Ce 3+ spin state The pumping dynamics of the ground-state spin state was revealed in the following way. A finite train of circularly polarized laser pulses (the duration of the pulse is 100 fs) was shot on the single Ce 3+ centre. The train contained 140 pulses with the repetition rate 2.5 MHz. The average laser power within the train was 50 μW at the entrance aperture of the microscope objective lens. After each pulse train, the cerium ion spin was allowed to relax to thermal equillibrium for 50 ms. After that, the excitation of the ion with the finite pulse train was repeated and the signals obtained for each pulse train were averaged. The resulting signal was fitted with an exponential decay function multiplied by two step-functions (step-up and step-down) in order to simulate the beginning and the end of the excitation pulse train. Implantation of cerium ions YAG crystals were implanted in EIKO FIB with accelerating voltage 100 kV. Ions were extracted from the liquid metal ion source Ce-Si-Au. Ions were separated with built-in Wien filter so that Ce 3+ were implanted with the energy of 300 keV. With the simulations performed in the SRIM software, we obtain penetration depth of 62 nm with straggle of 18 nm. Crystal was implanted with pattern of dots with fluences of 10 11 cm −2 and 2 × 10 12 cm −2 . This corresponds to ~10 3 and 2 × 10 4 ions implanted per spot. In order to activate the implanted ions, thermal annealing was performed in argon atmosphere at 1,100 °C for 1 h. The activation yield was estimated by comparing the brightness of the implanted spots with the brightness of a single native cerium ion. How to cite this article: Siyushev, P. et al. Coherent properties of single rare-earth spin qubits. Nat. Commun. 5:3895 doi: 10.1038/ncomms4895 (2014).